Direct measurement of dysprosium(III)˙˙˙dysprosium(III) interactions in a single-molecule magnet Lanthanide compounds show much higher energy barriers to magnetic relaxation than 3d-block compounds, and this has led to speculation that they could be used in molecular spintronic devices. Prototype molecular spin valves and molecular transistors have been reported, with remarkable experiments showing the influence of nuclear hyperfine coupling on transport properties. Modelling magnetic data measured on lanthanides is always complicated due to the strong spin–orbit coupling and subtle crystal field effects observed for the 4f-ions; this problem becomes still more challenging when interactions between lanthanide ions are also important. Such interactions have been shown to hinder and enhance magnetic relaxation in different examples, hence understanding their nature is vital. Here we are able to measure directly the interaction between two dysprosium(III) ions through multi-frequency electron paramagnetic resonance spectroscopy and other techniques, and explain how this influences the dynamic magnetic behaviour of the system. Fascinating physics has been observed in lanthanide-based molecules ranging from single nuclear spin detection and manipulation [1] , [2] , blocking of magnetization at unprecedentedly high temperatures for a molecule [3] , [4] , magnetic memory in chiral systems with a non-magnetic ground state [5] , [6] and energy barriers for loss of magnetization, U eff , an order of magnitude higher than observed for polymetallic d-block cages [7] , [8] . A diverse range of applications has been envisioned for lanthanide (Ln) containing molecules, including use as qubits for quantum information processing [9] , [10] and prototype devices such as molecular spin valves [11] and transistors [1] have been reported. These advances have been very rapid since the initial report that a terbium phthalocyanine compound could function as a single-molecule magnet (SMM) [12] . The SMM behaviour observed for Ln complexes is due to the large magnetic anisotropy of the individual ions, caused by strong spin–orbit coupling and the crystal field (CF) effects due to the ligand environment [13] , [14] . Other interactions, for example intermolecular effects, often favour efficient quantum tunnelling of magnetization at zero external field, and this factor can mean little magnetic hysteresis is seen even in compounds with very large U eff [13] . When considering polymetallic Ln complexes, the situation becomes even more complicated. Radical bridging ligands can provide a strong magnetic exchange pathway between two lanthanide ions, leading to magnetic hysteresis at 14 K [3] , [4] . In other compounds weak Ln···Ln interactions can shift the zero-field quantum tunnelling step to a finite field, known as exchange biasing [15] , with different effects on cryogenic magnetization curves depending on the sign of the exchange [16] , [17] or even mask single-ion slow relaxation modes [18] . More frequently, however, Ln···Ln interactions increase quantum tunnelling rates, leading to apparently lower U eff values when compared with paramagnetic Ln ions doped into a diamagnetic lattice [8] , [17] , [19] . Understanding how Ln···Ln interactions can have such different and seemingly contradictory influences is important for improving the performance of Ln SMMs. Understanding such interactions in polymetallic molecular Ln complexes is far from trivial. Part of this problem is that bulk magnetic measurements provide only indirect evidence of weak Ln···Ln interactions which can be difficult to distinguish from other contributions to the low energy physics, for example, CF effects, intermolecular interactions, impurities. In this work we study a {Dy 2 } complex where we can spectroscopically measure a Dy(III)···Dy(III) interaction that quenches SMM behaviour. We combine magnetic measurements, electron paramagnetic resonance (EPR) spectroscopy, ab initio calculations and far-infrared (FIR) spectroscopy to develop a simple model to describe the magnetic interaction in a Dy···Dy pair, and provide design criteria for when this interaction will lead to exchange biasing, and when it will lead to collapse of the SMM behaviour. Synthesis and structure Hydrated lanthanide nitrate Ln(NO 3 ) 3 · n H 2 O and 8-hydroxyquinoline (hqH) were combined in a 1:2.5 mole ratio and heated to reflux in MeOH for 3 h. Slow evaporation of this solution gave yellow block-shaped X-ray quality single crystals in a yield of 52–75%. Characterization by single crystal X-ray diffraction revealed an asymmetric lanthanide dimer with formula [hqH 2 ][Ln 2 (hq) 4 (NO 3 ) 3 ]·MeOH (Ln=Y III , 1 ; Tb III , 2 ; Dy III , 3 ; Ho III , 4 ; Er III , 5 ; Yb III , 6 and Lu III , 7 ; see Methods, Supplementary Tables 1 and 2 and Supplementary Data 1–7 ). Compounds 1 – 7 are isostructural, crystallizing in the monoclinic space group P2 1 /c ( Fig. 1a ; see Methods and Supplementary Tables 3–5 ). We focus on 3 as it has the most interesting magnetic properties. The dimer consists of two Dy(III) ions, three nitrate anions and four 8-quinolinolate ligands, crystallizing with a protonated 8-hydroxyquinolinium counter-cation and a molecule of MeOH. Dy(1) is bound by three bridging 8-quinolinolate ligands and a single chelating 8-quinolinolate ligand, generating an N 4 O 4 coordination environment with a bicapped trigonal prism geometry, subsequently referred to as the ‘hq pocket’ ( Fig. 1a ). The Dy(2) site binds to three chelating nitrate anions and the O-atoms from three bridging quinolinate ligands, yielding a highly distorted O 9 environment subsequently referred to as the ‘NO 3 pocket’. The eight-coordinate hq pocket is significantly smaller than the nine-coordinate NO 3 pocket: the volumes defined by the donor atoms are 130 and 140 Å 3 , respectively. 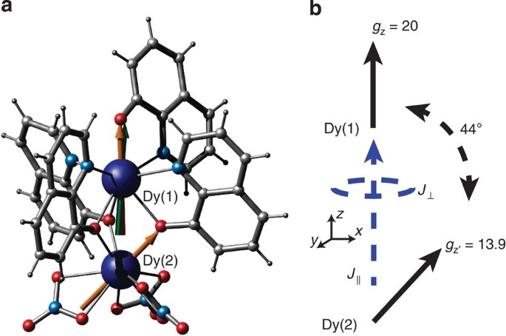Figure 1: Structural analysis. (a) Crystal structure of3. Scheme: Dy, blue; N, light blue; O, red; C, grey; H, dark grey. Orientation of the principal magnetic axes for Dy(1) and Dy(2) in the ground Kramers doublet fromab initiocalculations shown as orange arrows and that for Dy(1) from electrostatic calculations as green arrow. (b) Schematic of the magnetic model for the EPR simulation. Relative projection of the principal magnetic axes for Dy(1) and Dy(2), along whichgz=20 and 13.9 for Dy(1) and Dy(2), respectively, and the anisotropic exchange interaction between the dysprosium pair. Figure 1: Structural analysis. ( a ) Crystal structure of 3 . Scheme: Dy, blue; N, light blue; O, red; C, grey; H, dark grey. Orientation of the principal magnetic axes for Dy(1) and Dy(2) in the ground Kramers doublet from ab initio calculations shown as orange arrows and that for Dy(1) from electrostatic calculations as green arrow. ( b ) Schematic of the magnetic model for the EPR simulation. Relative projection of the principal magnetic axes for Dy(1) and Dy(2), along which g z =20 and 13.9 for Dy(1) and Dy(2), respectively, and the anisotropic exchange interaction between the dysprosium pair. Full size image As the two coordination sites are different in compounds 1 – 7 , we can take advantage of the lanthanide contraction to dope paramagnetic ions into one or the other of the two pockets of the diamagnetic yttrium or lutetium compound, 1 and 7 respectively [20] . Crystallographic studies on 1:1 heterobimetallic Ln-Y compounds (see Methods, Supplementary Tables 6–8 and Supplementary Data 8–13 ) show that Lu III occupies the smaller hq pocket in Lu-Y, while for the Dy-Y compound there is a distribution between the two pockets as Y III and Dy III have similar ionic radii. Therefore for Dy III doped at a low level into 7 , hereafter {Dy@Lu 2 }, Dy III is in the NO 3 pocket, while for Dy III doped at a low level into 1 , hereafter {Dy@Y 2 }, Dy III is distributed evenly between the two pockets. Magnetic measurements The room temperature χ M T value for 3 (26.8 cm 3 K mol −1 ) is close to the expected value for two non-interacting Dy III ions and declines smoothly on cooling reaching a minimum at 5 K ( Fig. 2a ) due to the depopulation of the CF states. Below 5 K χ M T increases due to a weak ferromagnetic interaction between the paramagnetic centres. The low temperature magnetization versus applied magnetic field does not saturate at 1.8 K in a field of 7 T, indicating strong magnetic anisotropy ( Fig. 2a inset). 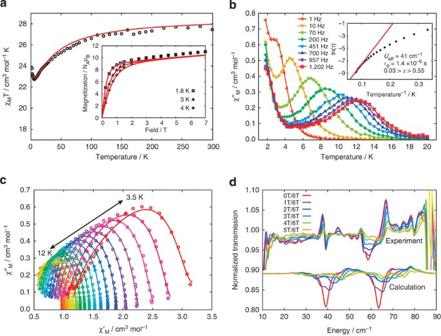Figure 2: Magnetic measurements. (a) ExperimentalχMT(T) andM(H,T) (inset) data (symbols) and best fits (red lines) for3. (b)χM′′(T) measured under a 1 kGHDCfield (1.55 G AC field) and Arrhenius treatment ofχM′′data for the high temperature process (inset) for {Dy@Y2}. (c) Cole-Cole plots (χM′′versusχM′) showing a single relaxation process above 3.5 K, solid lines are fits of the AC susceptibility data to a modified Debye function for {Dy@Y2}. (d) Normalized FIR transmission spectra at 9 K for3. Figure 2: Magnetic measurements. ( a ) Experimental χ M T ( T ) and M ( H , T ) (inset) data (symbols) and best fits (red lines) for 3 . ( b ) χ M ′′ ( T ) measured under a 1 kG H DC field (1.55 G AC field) and Arrhenius treatment of χ M ′′ data for the high temperature process (inset) for {Dy@Y 2 }. ( c ) Cole-Cole plots ( χ M ′′ versus χ M ′ ) showing a single relaxation process above 3.5 K, solid lines are fits of the AC susceptibility data to a modified Debye function for {Dy@Y 2 }. ( d ) Normalized FIR transmission spectra at 9 K for 3 . Full size image The dynamic magnetic behaviour of 3 was investigated through alternating current (AC) magnetic susceptibility measurements, performed both with a zero and a 1 kG applied direct current (DC) magnetic field. No frequency dependence was observed under zero DC field; whereas at 1 kG a small out-of-phase component is observed, but with no maximum in the temperature range 1.8–24 K ( Supplementary Fig. 1a–c ). By studying doped materials, we can show that the lacklustre dynamic behaviour observed in 3 is due to the effect of interactions between the Dy(III) ions. AC measurements on {Dy@Lu 2 } revealed only a small out-of-phase component below 3 K ( Supplementary Fig. 1d–f ), similar to that of the pure compound 3 . However the {Dy@Y 2 } analogue shows pronounced slow relaxation with frequency-dependent peaks in the out-of-phase susceptibility χ M ′′ to 12 K ( Fig. 2b,c and Supplementary Figs 2 and 3 ), when we use an optimal DC field of 1 kG ( Supplementary Fig. 2a ). Treating the highest temperature AC data with the Arrhenius model gives U eff =41 cm −1 and τ 0 =1.4 × 10 −6 s ( Fig. 2b inset); however, the lower temperature data is markedly nonlinear suggesting the onset of competing Orbach and Raman processes and this U eff value should be treated with some caution. Fitting the AC susceptibility data to a single Debye function reveals a single dominant relaxation path at higher temperatures (distribution parameter, α =0.03(1) at 12 K), with other pathways becoming competitive at lower temperatures ( α =0.55(2) at 3.5 K; Fig. 2c and Supplementary Fig. 3 ). From these observations we can determine that Dy(III) in the smaller hq pocket is an SMM, whereas Dy(III) in the larger NO 3 pocket is not. The SMM behaviour is quenched in the pure compound 3 due to intramolecular Dy···Dy interactions, vide infra. Ab initio calculations and FIR measurements Multi-configurational complete active space self-consistent field (CASSCF) calculations are the most accurate ab initio methods to rationalize the magnetic properties of lanthanide systems [6] , [8] , [15] , [21] , but they are not perfect and often require scaling to match absolute experimental values: this has been shown to be a result of neglected correlation energies and possible small structural changes at low temperatures [22] . We have performed such calculations on compound 3 with MOLCAS 7.8 (ref. 23 ; see Methods and Supplementary Table 9 ). Dy(III) has a 6 H 15/2 ground term, separated from the excited 6 H 13/2 term by roughly 4,000 cm −1 , and therefore we need only consider the ground multiplet for the magnetic properties. The CF removes the 16-fold degeneracy of the 6 H 15/2 multiplet giving eight Kramers doublets, which are linear combinations of m J =± 1 / 2 ···± 15 / 2 , where m J is the projection of J upon the axis of quantization. CASSCF calculations predict markedly different properties for the two Dy(III) sites in 3 ( Supplementary Tables 10 and 11 ), as expected given the different coordination environments. For Dy(III) in the hq pocket, the ground doublet is an almost pure m J =± 15 / 2 , as characterized by the calculated g z -value approaching 20 and g x and g y values close to zero. Its main magnetic axis lies along the Dy-O vector of the terminal 8-hydroxyquinolinolate ligand, which happens to be co-parallel with the Dy···Dy vector ( Fig. 1a ). Electrostatic optimization of the oblate m J =± 15 / 2 electron density [24] provides the same result (8.6° difference to CASSCF) and confirms that this orientation is due to the short terminal Dy-O bond of 2.248(3) Å ( c.f. 2.349(3)–2.384(3) Å for the bridging oxygen atoms), identical to the motif in the recently described homoleptic [Dy 3 (hq) 9 ] [25] . The first excited doublet is well separated from the ground state (~100 cm −1 ) and has dominant m J =± 13 / 2 character with its main magnetic axis ( g z ) almost colinear with that of the ground doublet. This is consistent with the observed SMM behaviour of {Dy@Y 2 }. For Dy(III) in the NO 3 pocket, the ground doublet has g -values of g z =16.42, g y =1.54, g x =0.05 ( Supplementary Table 11 ) and hence is not a pure m J =± 15 / 2 doublet. The first excited doublet is at only ~ 24 cm −1 , is strongly mixed and is misaligned with the ground doublet. This is consistent with {Dy@Lu 2 } not behaving as an SMM. The angle between the principal magnetic axes ( g z ) of the ground states for the two sites is calculated to be 44° by CASSCF ( Fig. 1a ). As the calculated CF splittings of the ground multiplet of Dy(III) in the NO 3 pocket lie squarely in the FIR region, we have used magnetic field-dependent FIR absorption spectroscopy [22] to measure them directly. Studies of compound 3 show two field-dependent bands at 39 and 59 cm −1 ( Fig. 2d and Supplementary Fig. 4 ) and therefore these are assigned as CF (as opposed to phonon) transitions. CASSCF predicts the first two CF transitions to be at 24 and 39 cm −1 . The agreement is remarkably good given that CF splittings for lanthanides can be several hundred wavenumbers. The ratio of the energy intervals is correct, and a simple scaling factor [22] of 1.6 (see above) gives the experimental energies ( Supplementary Table 12 ). The CASSCF results can be recast in the form of a set of CF parameters [26] . We have applied the FIR scaling factor to these parameters, and then used the scaled CF parameters ( Supplementary Table 13 ) to calculate magnetic observables and the magnetic transitions in the FIR spectra ( Fig. 2d ). This alone gives excellent agreement with experimental χ M T ( T ) from 5–300 K ( c.f. using unscaled CF parameters, Supplementary Fig. 5 ), but to simulate the low temperature χ M T ( T ) and M ( H ) data, we need to account for a weak exchange interaction. One way to simulate such thermodynamic data for orbitally degenerate ions is the Lines model [27] , which employs an isotropic exchange between the spin component of the angular momenta ( S = 5 / 2 for Dy(III); see Methods) and has been used previously to model interactions between lanthanides [15] , [28] . Employing this model with PHI [29] we find J Lines =+0.047(1) cm −1 , which gives excellent fits to both χ M T ( T ) and M ( H ) ( Fig. 2a ). EPR studies Weak exchange can be better defined by EPR spectroscopy, even between orbitally degenerate ions [30] , [31] , but such studies on lanthanide pairs are rare outside minerals, due to fast spin-lattice relaxation. Compound 3 , {Dy@Y 2 } and {Dy@Lu 2 } all give rich EPR spectra; the spectra of {Dy@Y 2 } and {Dy@Lu 2 } are very similar since in both cases we only see resonances for the Dy(III) ion in the NO 3 pocket. This is because Dy(III) in the hq pocket has an essentially pure m J =± 15 / 2 state, which is EPR silent and hence no g =20 resonance is observed. At low microwave frequencies (9.7, 24 and 34 GHz), the spectra of {Dy@Y 2 } and {Dy@Lu 2 } are dominated by an intense feature at g eff ≈14, which broadens at higher frequencies >130 GHz ( Fig. 3 and Supplementary Figs 6–8 ). There are other weaker features that match features from spectra of the pure compound 3 ( Fig. 3 and Supplementary Fig. 6 ). We simulate all spectra of the doped species with EasySpin [32] , using the effective spin formalism ( S eff = 1 / 2 ) with g x = g y =0.1, g z =13.9. The transverse g -values of 0.1 are arbitrarily small numbers and not measurable. The measured g z -value is similar to that calculated for the ground doublet of the NO 3 pocket by ab initio methods ( Supplementary Table 11 ) and is indicative of a strongly mixed ground state. 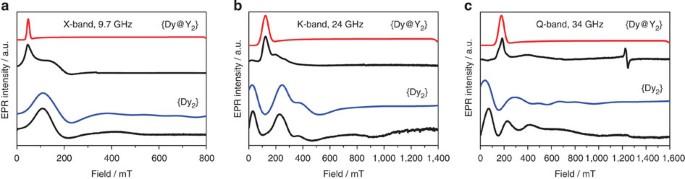Figure 3: EPR spectroscopy. X- (a), K- (b) and Q-band (c) experimental EPR spectra at 5 K (black traces) and simulated data for {Dy@Y2} (red traces) and3(blue traces). See text for simulation parameters. Figure 3: EPR spectroscopy. X- ( a ), K- ( b ) and Q-band ( c ) experimental EPR spectra at 5 K (black traces) and simulated data for {Dy@Y 2 } (red traces) and 3 (blue traces). See text for simulation parameters. Full size image The Dy···Dy exchange significantly perturbs the EPR spectra of compound 3 measured at lower frequencies (3.9, 9.7, 24 and 34 GHz) with multiple resonances observed ( Fig. 3 and Supplementary Fig. 9 ). For example, the 24 GHz spectrum of 3 has a resonance close to zero field; hence a splitting has been introduced equal to the microwave energy of ~0.8 cm −1 . The high-frequency EPR spectra are much broader, and therefore less sensitive to weak exchange interactions ( Supplementary Fig. 10 ). As an initial approach to modelling the EPR spectra of the coupled system, we can of course use the same approach employed for the fitting of the thermodynamic magnetic data, viz. the Lines model with scaled ab initio CFPs. Simulations of the low-frequency EPR spectra using the isotropic Lines exchange parameter (extracted from fitting the magnetometry data) yield some features of the spectra ( Supplementary Fig. 11 ), however, it is clear that the simulations are far from perfect. It is also clear from the spectra on doped samples that while the ab initio -calculated CFPs provide a decent approximation to the ground states, they are not a perfect starting point for examining the exchange interaction (that is, we must get the description of the individual sites correct before tackling the exchange interaction). Unfortunately due to the low symmetry of both pockets in this molecule, no reduction in the number of allowed CFPs can be made and therefore we are left with 27 parameters to describe each pocket. Clearly this problem is over-parameterised and it would not be feasible to find a unique solution. Therefore, a much simpler approach to simulating these spectra has been adopted, invoking a model of two effective spins, S eff = 1 / 2 . For the hq pocket we have g x = g y =0 and g z =20 from its EPR silent nature, SMM behaviour and ab initio calculations. For the NO 3 pocket, we have g z =13.9 from multi-frequency EPR spectroscopy on doped materials, and we take g x = g y =0.1. As both sites are axial in this model, we need only consider the relative orientation of the local z axes, which we fix at the ab initio -calculated angle of 44° ( Fig. 1b ). We define the molecular coordinate frame as that of the hq pocket (where z is along the g z vector of Dy(1) in the hq pocket, coincident with the Dy···Dy vector, and the two g z vectors define the zx plane). We can then use the Hamiltonian [1] to simulate the EPR spectra, where the only variables are the components of the anisotropic J -matrix. No agreement could be found for an isotropic J . The next simplest model has an axially symmetric J -matrix, where we set the principal component, J || , along the Dy···Dy vector ( Fig. 1b ). Using [1] we can model the EPR spectra of 3 with only two free variables, and we find excellent fits with J ⊥ =+0.525 cm −1 and J || =+1.52 cm −1 ( Fig. 3 and Supplementary Figs 9 and 10 ). This is a ferromagnetic interaction, consistent with the low temperature rise in χ M T ( T ). The spectra are not reproduced by a simple dipolar model ( =, , all other ; ) hence there is a significant exchange contribution, although we note that J || is very similar in magnitude to . With an accurate knowledge of the low energy eigenstates of our system, we are able to explain the lack of SMM behaviour in compound 3 . From the coupled S eff = 1 / 2 model used to simulate the EPR spectra, in zero field we have a ground doublet with wavefunctions ψ 1 =|↑↑› and ψ 2 =|↓↓› due to the ferromagnetic exchange. The two excited states are singlets at ~1 and ~2 cm −1 , which are the symmetric and antisymmetric linear combinations and , respectively ( Fig. 4 ). The average transition matrix elements (average of x , y and z magnetic transition probability) between the ground doublet wavefunctions vanish in zero field and no direct relaxation is possible. Even if we take into account the experimental perturbations, such as intermolecular dipole and hyperfine fields, direct magnetic relaxation between the two components of this doublet are unlikely due to this involving a flip of both moments. On the other hand, the average transition matrix elements between these doublet states and both the excited singlets are large, ~4 μ B 2 , indicating that relaxation processes involving these excited states are readily available. Given the small energy gaps to these excited states, they present an extremely efficient method for the reorientation of magnetization and thus explain the lack of any significant out-of-phase component in the AC susceptibility of 3 in zero field. 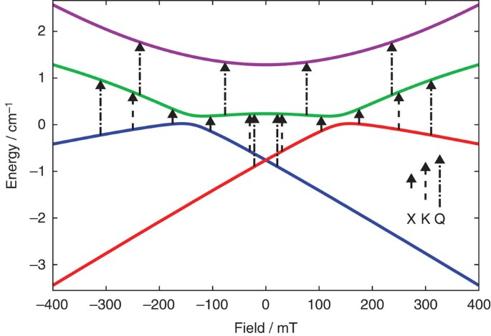Figure 4: Lowest energy states. All states in the EPR model for3, calculated as a function of magnetic field coincident with the principal axis of Dy(1). Blue line,ψ1; red line,ψ2; green line,ψ3; purple line,ψ4(see text). Arrows correspond to the EPR resonances observed for this orientation. Figure 4: Lowest energy states. All states in the EPR model for 3 , calculated as a function of magnetic field coincident with the principal axis of Dy(1). Blue line, ψ 1 ; red line, ψ 2 ; green line, ψ 3 ; purple line, ψ 4 (see text). Arrows correspond to the EPR resonances observed for this orientation. Full size image In a non-zero magnetic field, the situation is more complicated due to the anisotropic magnetic nature of the system. To illustrate our point we will discuss the case where the magnetic field is coincident with the principal axis of Dy(1) (as in Fig. 4 ). As the magnetic field is increased from zero, the component of the doublet that is destabilized by the field begins to strongly mix with the first singlet excited state. This mixing causes an avoided crossing between ψ 1 or ψ 2 and ψ 3 between | B |=100–150 mT and therefore significantly increases the average transition matrix elements between the two components of the doublet to a maximum value of ~2.4 μ B 2 at | B |=200 mT. Thus, in an applied DC magnetic field further relaxation pathways become available for the magnetization vector, therefore meaning that the applied field does not quench fast relaxation modes. For low microwave frequencies the EPR transition energies are on the scale of the exchange-induced splitting and even of the avoided crossing, hence these EPR experiments are directly measuring the probabilities and energies associated with the magnetic relaxation processes (see allowed EPR transitions marked on Fig. 4 ). The origin of these many efficient relaxation pathways is the non-colinearity of the principal axes of the Dy III ions. If we consider a scenario where the tilt angle of 44° between the two g z vectors is removed, but the exchange remains unchanged, the situation changes considerably. In zero field, while the average transition matrix elements between the ground doublet wavefunctions remains zero, the average transition matrix elements between these states and the excited singlets are now very small, on the order of 10 −3 μ B 2 , indicating that zero-field relaxation in this case would be hindered. With the application of a magnetic field along the easy axis ( Supplementary Fig. 12 ) the avoided crossings are no longer present, which implies that mixing between the ground doublet and the excited states does not occur and does not induce any transition matrix element between the components of the ground doublet. Therefore this hypothetical compound would be expected to show slow magnetic relaxation in zero field. Compound 3 shows very different physics from the exchange bias type of compounds, originally described by Wernsdorfer et al. [33] , and also seen in {Dy 2 } complexes [16] , where a remnant magnetization is present in the open hysteresis loops; a feature not observed here because of rapid zero-field relaxation. The hypothetical compound where the tilt angle is 0° may possibly show the characteristic QTM steps at the crossing points in Supplementary Fig. 12 once all perturbations are included and therefore we conclude that it is also the non-colinearity in 3 which distinguishes this compound from those of the exchange bias type. With the nature of the anisotropic magnetic exchange determined exactly by EPR spectroscopy, we are in a unique position to compare this with the magnetic exchange approximated by the Lines approach. Comparing the lowest four states obtained from EPR spectroscopy ( Fig. 4 ) to those of the Lines model used for fitting the magnetic susceptibility ( Supplementary Fig. 13 ), it is obvious that there are certain similarities. At zero field, the ground pseudo-doublet of the EPR model has g z ~34, which is identical to that of the Lines model of g z ~34, and the gap to the first excited state for the EPR model is ~1 cm −1 , also similar to that of the Lines model (~0.7 cm −1 ). It is also clear that the Lines approach yields two pseudo-doublets, whereas the excited states of the EPR model are singlets; this is a result of the anisotropic nature of the exchange interaction; such an interaction being excluded by the Lines approach. The high field limits of the two models are very similar, as would be expected due to the field ‘decoupling’ the individual moments in both cases (Paschen–Back effect). It is in the intermediate field regimes where the differences are most apparent, where we observe a number of avoided crossings in the EPR model and none in the Lines model. Intramolecular magnetic interactions between lanthanides are known to strongly influence magnetic relaxation. Here we can quantify this interaction, and demonstrate that it is the angle between the principal anisotropy axes and the associated magnetic exchange that has the effect of quenching the SMM behaviour in this dimetallic compound. Although the ferromagnetic exchange interactions lead to a highly magnetic ground state, the local transverse moment due to the asymmetric nature of the dimer makes relaxation very efficient. Many other {Dy 2 } complexes are reported to be SMMs [14] ; in every {Dy 2 } SMM where the orientation of the anisotropy axes is known, either from symmetry or calculation, they are parallel. In these cases, the Dy···Dy interaction is still present, but as it does not induce a transverse magnetic field at either Dy site, it does not destroy the barrier to magnetization reversal. This gives the design criterion that the magnetic moments of individual spins should be aligned parallel within polymetallic lanthanide SMMs to enhance measurable magnetization retention at zero field. Synthetic methods Compounds 1 – 6 were synthesized according to the following general method. To a solution of Ln(NO 3 ) 3 · n H 2 O (0.6 mmol), where Ln=Y III , Tb III , Dy III , Ho III , Er III , Yb III or Lu III , in MeOH (20 ml) was added 8-hyxdroxyquinolinoline (hqH; 220 mg, 1.5 mmol). The solution was then refluxed for 3 h and subsequently filtered. Yellow block crystals were collected after 24 h of slow evaporation crystallization for Y ( 1 ), Tb ( 2 ), Dy ( 3 ), Ho ( 4 ), Er ( 5 ), Yb ( 6 ) and Lu ( 7 ) ( Supplementary Table 1 ). The magnetically dilute samples, {Dy @ Y 2 } and {Dy @ Lu 2 }, were obtained by combining accurately measured amounts of Dy(NO 3 ) 3 · n H 2 O and Y(NO 3 ) 3 · n H 2 O or Lu(NO 3 ) 3 · n H 2 O in a 5:95 molar ratio, following the procedure above. The 1:1 mixed-metal systems were prepared by reacting Ln(NO 3 ) 3 · n H 2 O (where Ln=Tb III , Dy III , Ho III , Er III , Yb III and Lu III ) with Y(NO 3 ) 3 · n H 2 O in a 1:1 molar ratio using the procedure described above. Crystallography The crystallographic data for 2 was collected on a Bruker Prospector CCD diffractometer with CuK α radiation ( λ =1.5418 Å). The crystallographic data for 3 – 5 were collected on an Oxford SMART CCD diffractometer with MoK α radiation ( λ =0.71073 Å). The data collection for 7 was carried out on Agilent SUPERNOVA diffractometer with MoK α radiation ( λ =0.71073 Å). The data for 1 and 6 were collected on a Rigaku Saturn724+ diffractometer (synchrotron, λ =0.68890 Å) at the I19 beamline at the Diamond Light Source, UK. The structures were solved by direct methods and refined on F 2 using SHELXTL. Electron paramagnetic resonance X-band ( ~ 9.7 GHz) and Q-band ( ~ 34 GHz) EPR spectra were recorded with a Bruker EMX580 spectrometer, while S-band ( ~ 3.9 GHz) and K-band ( ~ 24 GHz) EPR spectra were recorded with a Bruker Elexsys580 spectrometer. The data were collected on polycrystalline powders in the temperature range 5–30 K using liquid helium cooling. High-frequency EPR spectra (260–380 GHz) were recorded in Stuttgart on a home-built spectrometer. Its radiation source is a 0–20 GHz signal generator (Anritsu) in combination with an amplifier–multiplier chain (VDI) to obtain the required frequencies. It features a quasi-optical bridge (Thomas Keating) and induction mode detection. The detector is a QMC magnetically tuned InSb hot electron bolometer. The sample is located in an Oxford Instruments 15/17T cryomagnet equipped with a variable temperature insert (1.5–300 K). Spectral simulations were performed using the EasySpin 4.5.5 simulation software. Magnetometry The magnetic properties of polycrystalline samples of 2 – 6 were investigated in the temperature range 1.8–300 K with a Quantum Design MPMS-XL7 SQUID magnetometer equipped with a 7 T magnet. The samples were ground, placed in a gel capsule and fixed with a small amount of eicosane to avoid movement during the measurement. The data were corrected for the diamagnetism from the gel capsule and the eicosane, with the diamagnetic contribution of the complexes calculated from Pascal’s constants. AC susceptibility measurements were performed with an AC field of 1.55 G oscillating at frequencies between 1 and 1,400 Hz. Far infrared FIR spectra were recorded using a Bruker 113v FTIR spectrometer equipped with a mercury light source. For the detection we used an Infrared Laboratories pumped Si bolometer (operating temperature 1.5 K). For samples we used 10 mm pressed powder pellets. The samples were placed in an Oxford Instruments Spectromag 4000 optical cryostat allowing fields up to 8 T and temperatures down to 1.8 K. The sample holder permitted in situ change between an aperture and the sample, which allowed recording absolute transmission spectra. CASSCF calculations The CASSCF calculations were performed with MOLCAS 7.8 using the geometry as elucidated with X-ray crystallography. All calculations considered the individual Dy III ions independently, where the ion not in focus was replaced by the diamagnetic Lu III . All calculations were of the complete active space type where the 4f 9 configuration of Dy III was modelled with nine electrons in seven orbitals CAS(9,7), using the RASSCF module. The basis sets for these calculations were taken from the ANO-RCC library, where the paramagnetic ion was of VTZP quality, the first coordination sphere of VDZP quality and all other atoms of VDZ quality. Supplementary Table 9 details the states included in the RASSCF and RASSI modules. The RASSI module was used to calculate the g-tensors for the 6 H 15/2 multiplet [34] and SINGLE_ANISO was used to generate a complete set of CF parameters from the ab initio -calculated spin–orbit eigenstates [35] . CF and lines models The CF parameters (CFPs) were treated as explained in the main text, and the reference frame rotations were optimized to reproduce the mutual orientations from the ab initio calculations ( Supplementary Table 13 ). These were fixed while the exchange interaction was fitted to the magnetic data. The following Hamiltonian was used in the | J , m J › basis for each Dy III ion, where the exchange term acts on the true spins ( S = 5 / 2 ) for each Dy III and the term was evaluated using a Clebsch–Gordan decomposition. θ k are the operator equivalent factors for Dy III in the | J , m J › basis, g J is the Landé g -factor for the 6 H 15/2 term of Dy III and is equal to 4 / 3 , I is the identity matrix and J Lines is the exchange parameter. Note that the operators are expressed in the local coordinate frame of each Dy III ion, using the given Euler angles. EPR simulation with the Lines model Using exactly the same Hamiltonian as above, the EPR was simulated in a non-perturbative manner with PHI. The EPR absorption spectrum was calculated at discrete field points using the following equation, where and are the Zeeman Hamiltonians for the components of the perpendicular microwave magnetic field, E i and E j are the energies for the states | i › and | j › (eigenstates of the above Hamiltonian), respectively, Z is the partition function and η is the linewidth expressed in energy units. As the linewidth is evaluated in frequency space, there is no need for the frequency-field conversion factor. The absorption spectrum was summed over a large number of orientations on a hemisphere using the Zaremba–Conroy–Wolfsberg spherical integration scheme [36] . The first derivative of the absorption spectrum was then obtained to yield the spectral simulations. Accession codes: The X-ray crystallographic coordinates for structures reported in this study have been deposited at the Cambridge Crystallographic Data Centre (CCDC), under deposition numbers CCDC 1011262–1011274. These data can be obtained free of charge from The Cambridge Crystallographic Data Centre via www.ccdc.cam.ac.uk/data_request/cif, (or from the Cambridge Crystallographic Data Centre, 12 Union Road, Cambridge CB21EZ, UK; fax: (+44)1223-336-033; or deposit@ccdc.cam.ac.uk). How to cite this article: Pineda, E. M. et al. Direct measurement of dysprosium(III)···dysprosium(III) interactions in a single-molecule magnet. Nat. Commun. 5:5243 doi: 10.1038/ncomms6243 (2014).